Blimp1 regulates the transition of neonatal to adult intestinal epithelium In many mammalian species, the intestinal epithelium undergoes major changes that allow a dietary transition from mother's milk to the adult diet at the end of the suckling period. These complex developmental changes are the result of a genetic programme intrinsic to the gut tube, but its regulators have not been identified. Here we show that transcriptional repressor B lymphocyte-induced maturation protein 1 (Blimp1) is highly expressed in the developing and postnatal intestinal epithelium until the suckling to weaning transition. Intestine-specific deletion of Blimp1 results in growth retardation and excessive neonatal mortality. Mutant mice lack all of the typical epithelial features of the suckling period and are born with features of an adult-like intestine. We conclude that the suckling to weaning transition is regulated by a single transcriptional repressor that delays epithelial maturation. Mice are born with immature intestinal epithelium that is optimally adapted to the diet of mother's milk. To process the high-fat diet, which contains lactose as a principal source of carbohydrates, enterocytes are specialized to metabolize fatty acids and express high levels of lactase on the brush border [1] . Enterocytes in the distal intestine of suckling rodents as well as of humans can be recognized by the presence of large vacuoles, important for transport of maternal immunoglobulins and other macromolecules across the epithelial barrier [2] , [3] . At birth, mouse intestinal epithelium does not contain crypts. Instead, proliferative cells are restricted to the epithelium between the villi, so-called intervillus pockets [4] . Around 1 week after birth, the intervillus epithelium reshapes to form crypts, which gradually increase in size and number within the next two postnatal weeks. [4] Paneth cells appear coincidental with crypt formation [5] . They reside at the crypt base interspersed with stem cells and are specialized to secrete antimicrobial proteins such as the α-defensins (cryptdins) and lysozyme [6] , [7] . The intestinal epithelium undergoes major structural and biochemical changes at the suckling to weaning transition to adapt to solid foods that contain mainly carbohydrates [1] . One important example of this adaptation is the switch of brush border disaccharidase expression from lactase to sucrase isomaltase [8] . Sucrase isomaltase is an enzyme specialized in digestion of complex carbohydrates present in solid food. After weaning, the intestine is less permeable for the luminal content and the enterocyte vacuolization is absent. This loss in absorptive capacity is compensated by an increase in the absorptive surface because of intestinal growth and a better-developed brush border. It was initially believed that the epithelial changes during the suckling to weaning transition might be secondary to the major changes in diet and gut microflora in this period [9] , [10] , [11] , [12] . Changes in circulating hormones in the developing neonate such as glucocorticoids have been pursued as an alternative regulatory mechanism [13] , [14] . However, although such external factors may influence the timing of the transition, a series of careful experiments have established that intestinal epithelial maturation is a process that is intrinsic to the gut tube and occurs independent of external factors. For example, when embryonal intestinal segments were transplanted into adult animals, they developed normally and maintained the correct positional information, both in terms of crypt–villus structure and patterning along the longitudinal axis [15] , [16] , and showed a normal suckling to weaning transition [17] . These experiments have clearly established that appropriate intestinal epithelial development is independent of luminal signals and of the hormonal contexts of pregnancy or the early postnatal period. Instead it is regulated by a genetic programme that is intrinsic to the gut tube and is specified early in endodermal development. B-lymphocyte-induced maturation protein 1 (Blimp1) (gene name Prdm1 ) is a transcriptional repressor that has an important role in many embryonic and adult tissues. For example, Blimp1 is critical for the maintenance of germ cell fate by repressing a somatic programme that is adopted by neighbouring cells [18] . In B cells, Blimp1 mediates the terminal differentiation into immunoglobulin-secreting plasma cells by repressing the mature B-cell gene expression programme [19] . In skin, it functions to repress the sebaceous gland cell differentiation programme in sebaceous gland precursor cells of the hair follicle [20] . Blimp1 uses different modes of repression that depend on the cellular context and recruitment of various corepressors such as members of the Groucho family of repressors, [21] histone methyltransferases [22] , [23] and histone deacetylases [24] . In this study we observed that Blimp1 is highly expressed in the postnatal intestinal epithelium and found that expression is almost completely lost at the suckling to weaning transition. We studied the role of Blimp1 in the intestinal epithelium in mice with intestine-specific deletion of Blimp1 and suggest that this transcriptional repressor delays epithelial maturation. Blimp1 expression in development and the neonatal intestine Blimp1 is expressed in the developing gut endoderm from embryonic day 9 (E9) until birth [25] . We examined expression of Blimp1 in the intestinal epithelium and made the surprising observation that there is a sharp decline in Blimp1 expression in the third postnatal week ( Fig. 1 ). At E19, Blimp1 expression showed a gradient with low expression in the intervillus pockets and high expression in the epithelial cells on the villi. At postnatal day 7 (P7), intervillus pockets were Blimp1-negative ( Supplementary Fig. S1 ). Between the second and third postnatal week, expression of the protein was gradually lost and finally confined to only a few cells at the villus tip in adult animals. We conditionally deleted Blimp1 from the adult intestinal epithelium using Cyp1a1CreBlimp1 fl/fl mice to examine whether Blimp1 expression at the villus tip might have some function in, for example, exfoliation of epithelial cells. We did not observe any phenotype in these mice that were killed at different time points after deletion of Blimp1, despite the confirmation of successful and stable deletion ( Supplementary Fig. S2 ). In order to examine the role of Blimp1 during development, we crossed the Blimp1 fl/fl mouse with the VillinCre mouse strain, in which the villin promoter drives the expression of Cre recombinase in the intestinal epithelium from E14.5 throughout the lifetime of the mouse [26] . 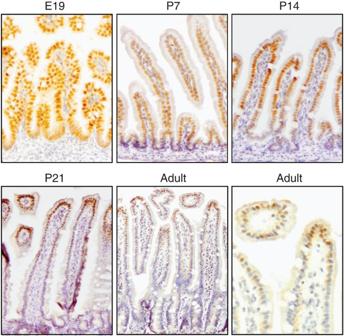Figure 1: Blimp1 is expressed until the suckling to weaning transition in the intestinal epithelium of the mouse. Immunohistochemistry shows nuclear localization of Blimp1 in the small intestinal epithelium, which becomes restricted to the upper part of the villus around day 21 and finally only marks a few cells at the villus tip in adult mice (arrows in enlargement). Original magnifications: ×200 and ×800 for magnification. Figure 1: Blimp1 is expressed until the suckling to weaning transition in the intestinal epithelium of the mouse. Immunohistochemistry shows nuclear localization of Blimp1 in the small intestinal epithelium, which becomes restricted to the upper part of the villus around day 21 and finally only marks a few cells at the villus tip in adult mice (arrows in enlargement). Original magnifications: ×200 and ×800 for magnification. Full size image Postnatal mortality and reduced growth in Blimp1 mutant mice In fourth generation crosses of the VillinCre transgene and Blimp1 fl/+ mutant mice, all pups were VillinCre -positive and Blimp1 fl/fl mice were born with the expected Mendelian ratio. In three consecutive litters from VillinCre + Blimp1 +/fl parents genotyped at P0, we obtained 23 pups of which 5 were Blimp1 fl/fl (mutant), 5 were Blimp1 +/+ (wild type) and 13 were Blimp1 +/fl (heterozygous). We noted that many of the mice were lost in the first postnatal week. In five consecutive litters from VillinCre + Blimp1 +/fl parents genotyped at the moment of killing at P7, 55 pups were born, but only 46 survived until P7. At P7, only 4.3% of the surviving mice were Blimp1 mutant rather than the expected 25%, indicating that the excess mortality occurred in the Blimp1 mutant animals. Indeed, whereas weight of wild type and Blimp1 mutant animals was similar at E17.5 and at birth ( Fig. 2a ), surviving Blimp1 mutant animals displayed severe growth retardation in the postnatal phase ( Fig. 2a,b ). At P7, wild-type mice had an average weight of 4.4±0.12 g (mean and standard error, n =30) compared with only 2.74±0.15 g ( n =11, P <0.0001, Student's t -test) for littermate Blimp1 mutant animals, a weight reduction of 38%. This growth defect persisted until adult life ( Fig. 2a ). We focused our histological analyses on P7 as it represents the phase of the suckling period when all specialized features of the neonatal intestine are fully developed [27] . We found near-complete deletion of Blimp1 along the entire longitudinal axis of the small intestine ( Fig. 3a ). In the ileum, we observed a few small regions of epithelium that still contained some Blimp1-positive cells. 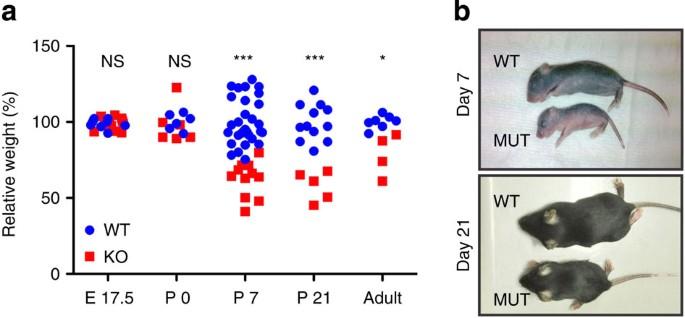Figure 2: Growth retardation in mice with intestinal epithelial deletion of Blimp1. (a) Relative weight of Blimp1 mutant and control littermates at different ages. (b) Representative images of Blimp1 mutant and control animals at P7 and P21 shows growth retardation of the mutants. NS, not significant; HET, heterozygote; MUT, mutant; WT, wild type. *P<0.05; ***P<0.001, Student'st-test. Figure 2: Growth retardation in mice with intestinal epithelial deletion of Blimp1. ( a ) Relative weight of Blimp1 mutant and control littermates at different ages. ( b ) Representative images of Blimp1 mutant and control animals at P7 and P21 shows growth retardation of the mutants. NS, not significant; HET, heterozygote; MUT, mutant; WT, wild type. * P <0.05; *** P <0.001, Student's t -test. 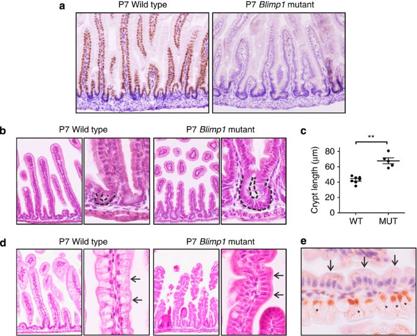Figure 3: Accelerated maturation of Blimp1 mutant intestinal epithelium. (a) Immunohistochemistry for Blimp1 shows efficient loss of Blimp1 from the intestinal epithelium. (b) In the proximal small intestine, there was a noticeably enhanced formation of crypts (dotted line) at P7 compared with the rudimentary crypts (dotted line) of the wild-type mice. (c) Average crypt depth in wild type (WT,n=7) and Blimp1 mutant (MUT,n=5) animals, average plus s.e. (d) In the distal small intestine of WT mice, enterocytes clearly showed the translucent cytoplasm that is typical for the presence of large cytoplasmic vacuoles that characterize this stage (arrows). These vacuoles were completely absent in Blimp1 mutant enterocytes (arrows). (e) A rare villus on which Blimp1 is only partially deleted clearly shows the difference in phenotype between Blimp proficient (brown nuclear staining, asterisks) and deficient cells (arrows). **P<0.01, Student'st-test. Original magnifications ×200 for overviews and ×800 for enlargements. Full size image Figure 3: Accelerated maturation of Blimp1 mutant intestinal epithelium. ( a ) Immunohistochemistry for Blimp1 shows efficient loss of Blimp1 from the intestinal epithelium. ( b ) In the proximal small intestine, there was a noticeably enhanced formation of crypts (dotted line) at P7 compared with the rudimentary crypts (dotted line) of the wild-type mice. ( c ) Average crypt depth in wild type (WT, n =7) and Blimp1 mutant (MUT, n =5) animals, average plus s.e. ( d ) In the distal small intestine of WT mice, enterocytes clearly showed the translucent cytoplasm that is typical for the presence of large cytoplasmic vacuoles that characterize this stage (arrows). These vacuoles were completely absent in Blimp1 mutant enterocytes (arrows). ( e ) A rare villus on which Blimp1 is only partially deleted clearly shows the difference in phenotype between Blimp proficient (brown nuclear staining, asterisks) and deficient cells (arrows). ** P <0.01, Student's t -test. Original magnifications ×200 for overviews and ×800 for enlargements. Full size image Blimp1 specifies morphological hallmarks of neonatal intestine Histological analysis of Blimp1 mutant versus littermate Blimp1 wild-type animals at P7 revealed striking differences in the morphology of the two genotypes. At P0, proliferating cells are localized in so-called intervillus pockets that will reshape to form crypts between the first and third postnatal weeks [28] . At P7, much of the intestinal epithelium in wild-type animals still lacked crypts, but early crypt formation can be observed ( Fig. 3b ). In Blimp1 mutants, crypt formation was accelerated ( Fig. 3b,c ). Average crypt depth was 43±1.7 μm (mean and standard error) in wild types ( n =7, >30 crypts counted per animal) compared with 68±3.9 μm in Blimp1 mutant mice ( n =5, >30 crypts counted per animal, P <0.01, Student's t -test). c-Myc and Sox9 are important regulators of the precursor cell phenotype in the crypts [29] , [30] . We therefore examined the expression of c-Myc and Sox9 in wild-type ( n =4) and Blimp1 mutant ( n =4) mice. We could not detect a clear difference in their expression ( Supplementary Fig. S3 ). Cdx2 has previously been found to regulate epithelial maturation when overexpressed in the intestinal epithelium [31] , but we found no difference in expression of Cdx2 between wild types and Blimp1 mutants ( Supplementary Fig. S3 ). Another striking difference in the histology of the mutant mice was the complete absence of the large vacuoles that normally characterize the enterocytes of the distal small intestine in neonatal animals until the third postnatal week ( Fig. 3d,e ). In addition, villi of mutant animals had a more serrated appearance typical for the adult intestine. Under higher magnification, intestinal enterocyte brush border seemed more developed. These features were further confirmed by electron microscopic (EM) imaging ( Fig. 4 ). In wild-type ( n =3) animals, EM showed the apical canalicular system ( Fig. 4a ) that feeds into the large cytoplasmic vacuoles ( Fig. 4b ), from the intestinal lumen at the apical side of the enterocyte. The large vacuoles were partially filled with mucous-like content. In Blimp1 mutant ( n =3) enterocytes, both the canalicular system and vacuoles were completely absent. EM also showed that the microvilli were much better developed in Blimp1 mutant animals ( Fig. 4c ). Thus, the microscopic and submicroscopic morphological differences between wild type and Blimp1 mutant animals were consistent with an accelerated maturation of the epithelium in mutant animals. 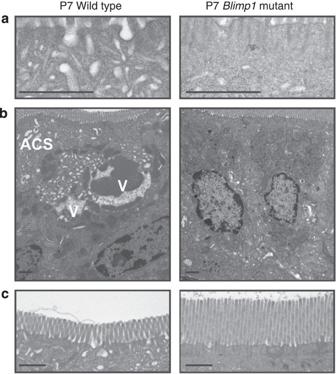Figure 4: Transmission electron microscopy shows loss of vacuoles and accelerated brush border development in Blimp1 mutants. (a) Image of the apical canalicular system of a wild-type (WT) mouse. Mutant (MUT) mice completely lack this system. (b) An image of a whole cell clearly shows how the apical canalicular system (ACS) feeds into large cytoplasmic vacuoles (Vs) in WT mice and that this system is absent in Blimp1 mutants. (c) An image of the brush borders of WT and MUT mice shows a much more developed brush border in mutant mice. Bars in left lower corners indicate 1 μm. Figure 4: Transmission electron microscopy shows loss of vacuoles and accelerated brush border development in Blimp1 mutants. ( a ) Image of the apical canalicular system of a wild-type (WT) mouse. Mutant (MUT) mice completely lack this system. ( b ) An image of a whole cell clearly shows how the apical canalicular system (ACS) feeds into large cytoplasmic vacuoles (Vs) in WT mice and that this system is absent in Blimp1 mutants. ( c ) An image of the brush borders of WT and MUT mice shows a much more developed brush border in mutant mice. Bars in left lower corners indicate 1 μm. Full size image Blimp1 is required to adapt enterocytes to the suckling period We further explored the differences between Blimp1 wild type and mutant animals at P7 exploiting microarray technology. This provided 254 differentially expressed genes with P <0.01 (false discovery rate was also 0.01) and gene pattern software revealed that Blimp1 mutant and wild-type animals grouped into two distinct clusters ( Fig. 5a ). This indicates a clear difference in expression patterns between Blimp1 mutants and wild types, but a high degree of similarity within the two different sample groups. Ingenuity software analysis showed that most of the changes were associated with metabolic pathways ( Fig. 5b ). Strikingly, the most upregulated gene in Blimp1 mutant animals ( Supplementary Data 1 ) is the brush border enzyme sucrase isomaltase. Sucrase isomaltase digests complex carbohydrates and the induction of its expression marks the transition of suckling to weaning-type epithelium in mice [32] . In the list of downregulated genes, we identified β-galactosidase, an enzyme that we found is specifically expressed in the sucking period when it localizes to the cytoplasmic vacuoles (see below). This β-galactosidase expression during the suckling period is likely involved in the cytoplasmic processing of lactose [33] , [34] . The Illumina array did not contain any probe set for the lactase gene, the major brush border enzyme involved in lactose metabolism, but we were able to confirm its downregulation at the protein level (see below). The net effect of this change is an inversed expression pattern in these disaccharidases. Blimp1 mutant animals express sucrase isomaltase long before its normal developmental onset, but have lost the expression of the two disaccharidases required for the digestion of lactose. Within the first five most upregulated genes were trehalase and adenosine deaminase , both of which normally follow the same developmental pattern as sucrase isomaltase [35] , [36] . This indicates that there is a general derepression of enzymes that should normally only be expressed after the suckling to weaning transition. 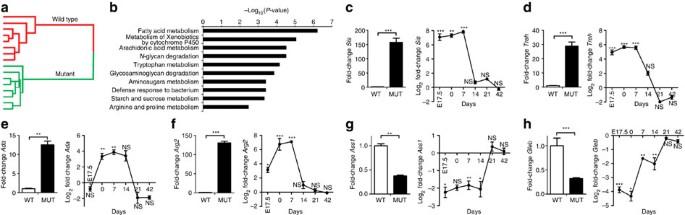Figure 5: A major metabolic shift towards the adult phenotype in Blimp1 mutant (MUT) mice at P7. (a) Cluster analysis of the individual mice on the gene array showed that the MUT animals group together and are a separate cluster from the wild-type (WT) mice. (b) Most of the pathways that are significantly altered in the MUT mice are metabolic pathways. (c–h) Real-time RT–PCR analysis of selected candidates from the significantly altered genes identified in the array. (c) Sucrase isomaltase (Sis), (d) trehalase (Treh), (e) adenosine deaminase (Ada), (f) arginase 2 (Arg2), (g) argininosuccinate synthetase 1 (Ass1), (h) β-galactosidase (Gleb). For each gene the fold difference at P7 is shown on the left and the Log2 fold differences at different time points on the right. For E17.5, P0 and 1, 2, 3 and 6 weeks the number of WT animals isn=5,n=3,n=7,n=5,n=7,n=8, respectively, whereasn=5,n=3,n=8,n=7,n=6 andn=10 for the MUT animals, respectively. *P<0.05; **P<0.01 and ***P<0.001, NS, not significant. Data were analysed using a two-way analysis of variance, mean and s.e. are shown. Figure 5: A major metabolic shift towards the adult phenotype in Blimp1 mutant (MUT) mice at P7. ( a ) Cluster analysis of the individual mice on the gene array showed that the MUT animals group together and are a separate cluster from the wild-type (WT) mice. ( b ) Most of the pathways that are significantly altered in the MUT mice are metabolic pathways. ( c – h ) Real-time RT–PCR analysis of selected candidates from the significantly altered genes identified in the array. ( c ) Sucrase isomaltase (Sis), ( d ) trehalase (Treh), ( e ) adenosine deaminase (Ada), ( f ) arginase 2 (Arg2), ( g ) argininosuccinate synthetase 1 (Ass1), ( h ) β-galactosidase (Gleb). For each gene the fold difference at P7 is shown on the left and the Log2 fold differences at different time points on the right. For E17.5, P0 and 1, 2, 3 and 6 weeks the number of WT animals is n =5, n =3, n =7, n =5, n =7, n =8, respectively, whereas n =5, n =3, n =8, n =7, n =6 and n =10 for the MUT animals, respectively. * P <0.05; ** P <0.01 and *** P <0.001, NS, not significant. Data were analysed using a two-way analysis of variance, mean and s.e. are shown. Full size image We also found changes in the metabolism of arginine, as arginase 2 was among the top upregulated genes, whereas argininosuccinate synthetase 1 was significantly downregulated. Arginine is a 'conditionally' essential amino acid, which is mainly essential during periods of growth and tissue repair. Arginine is therefore critical for the proper growth of a neonate, but milk contains too little arginine to sustain normal growth [37] . As the arginine precursors, proline and glutamine are abundant in milk, the small intestinal epithelium of many species generates arginine from proline during the suckling period [38] . As a result, the enterocytes of suckling animals and humans express high levels of argininosuccinate synthetase 1, which is required for a key intermediate step in arginine synthesis, by catalysing the conversion of citrulin to arginine [39] , [40] . At the same time, neonates do not express any arginase, which is only expressed after the weaning transition, resulting in low intestinal epithelial catabolism and a prominent role for the intestine in arginine production [41] , [42] . Blimp1 mutant mice showed an inversed expression of these two enzymes with derepression of arginase 2 expression and loss of argininosuccinate synthetase 1 expression. This is again a feature of inappropriate adult-like features of the epithelium in the mutant mice and will severely impair both arginine synthesis from milk and its distribution in the bloodstream. We confirmed the changes in the expression pattern of all of these genes by real-time RT–PCR in a time course analysis ( Fig. 5c–h ). The analysis showed that the difference between wild types and Blimp1 mutants was restricted to the suckling period when Blimp1 is actually expressed. We observed no significant differences in expression after the suckling to weaning transition, which is around P21. Moreover, we found that the changes in gene expression in Blimp1 mutant animals were already present at E17.5 ( Fig. 5c–h ). We next examined the expression of these differentially regulated genes at the protein level by performing immunohistochemistry for lactase, sucrase isomaltase, adenosine deaminase, trehalase, argininosuccinate synthetase 1 and β-galactosidase ( Fig. 6 ). This immunohistochemical analysis confirmed the observations made at the mRNA level. 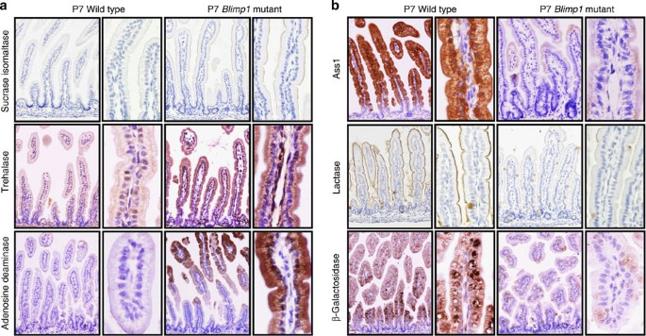Figure 6: Adult-type enzyme expression pattern in Blimp1 mutant (MUT) mice. Immunohistochemistry shows that (a) the adult-type enzymes sucrase isomaltase, trehalase and adenosine deaminase are aberrantly expressed in MUT mice. (b) In contrast, expression of suckling-period-specific enzymes such as argininosuccinate synthetase 1, lactase and β-galactosidase are lost. Note the localization of β-galactosidase to the cytoplasmic vacuoles in the wild-type animal. Original magnifications ×200 and ×800 for enlargements. Figure 6: Adult-type enzyme expression pattern in Blimp1 mutant (MUT) mice. Immunohistochemistry shows that ( a ) the adult-type enzymes sucrase isomaltase, trehalase and adenosine deaminase are aberrantly expressed in MUT mice. ( b ) In contrast, expression of suckling-period-specific enzymes such as argininosuccinate synthetase 1, lactase and β-galactosidase are lost. Note the localization of β-galactosidase to the cytoplasmic vacuoles in the wild-type animal. Original magnifications ×200 and ×800 for enlargements. Full size image Increased epithelial turnover time in Blimp1 mutant mice The epithelium of suckling animals has a considerably slower rate of turnover than that of adult animals. This has been especially well described in rats, in which migration of intestinal epithelial cells is four times faster in adults than in suckling rats [43] . To examine the rate of epithelial migration, Blimp1 mutant ( n =4) and wild type ( n =4) pups were injected with 7.5 mg kg −1 bromodeoxyuridine (BrdU) intraperitoneally at P4 and killed 5 days later at P9 to examine the migration of BrdU-labelled cells along the crypt–villus axis. As expected, the migration of epithelial cells to the villus tip was considerably slower in the suckling period than in the 3–5 days, typical for adult animals [44] . In wild-type animals, BrdU-positive cells reached only up to 61% of the length of the villi in 5 days. In contrast, in mutant mice, cells had travelled 98% of the villus length on average ( P <0.05, Student's t -test) in the same time frame of 5 days ( Fig. 7 ). In order to explain the difference in the rate of migration, the Blimp1 mutant animals should either have an increased number of precursor cells or an accelerated cell cycle. As we found no clear difference in the number of precursor cells between wild type and Blimp1 mutant animals, based on c-Myc- and Sox9-positive cells ( Supplementary Fig. S3 ), we examined whether the precursor cells could have a shortened cell cycle. To this end, we injected wild type and Blimp1 mutant animals with 7.5 mg kg −1 BrdU intraperitoneally at P7 and killed them 2 h later. We found that there was no difference in the number of precursor cells judged by staining with anti-Ki67 ( Fig. 7c ). However, an increase in the number of BrdU-positive cells in S phase was observed in Blimp1 mutant animals ( Fig. 7d ). In conclusion, the faster rate of epithelial migration in the mutant mice is sustained by an accelerated cell cycle of precursor cells. This represents yet another aspect of the premature maturation of the intestinal epithelium. 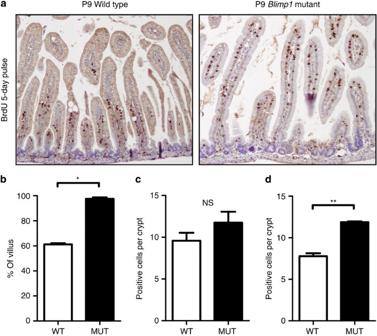Figure 7: Accelerated intestinal epithelial migration in Blimp1 mutant (MUT) animals. Animals were injected with BrdU at P4 and killed at P9 to examine the speed of epithelial migration along the crypt–villus axis. (a) Immunohistochemistry for BrdU in wild type (WT) and Blimp1 MUT animals. (b) In WT (n=5) animals, cells had migrated an average of 61% of the villus length compared with 98% in the MUT (n=5) animals. (c) Number of Ki67-positive cells per crypt (n=8 animals per group). (d) Number of BrdU-positive cells per crypt (n=2 animals per group). Average and s.e. value is shown, *P<0.05; **P<0.01, Student'st-test. NS not significant. Figure 7: Accelerated intestinal epithelial migration in Blimp1 mutant (MUT) animals. Animals were injected with BrdU at P4 and killed at P9 to examine the speed of epithelial migration along the crypt–villus axis. ( a ) Immunohistochemistry for BrdU in wild type (WT) and Blimp1 MUT animals. ( b ) In WT ( n =5) animals, cells had migrated an average of 61% of the villus length compared with 98% in the MUT ( n =5) animals. ( c ) Number of Ki67-positive cells per crypt ( n =8 animals per group). ( d ) Number of BrdU-positive cells per crypt ( n =2 animals per group). Average and s.e. value is shown, * P <0.05; ** P <0.01, Student's t -test. NS not significant. Full size image Blimp1 mutant mice show accelerated Paneth cell development Mice are born without Paneth cells, which start to appear in the first 2 weeks after birth, coincident with the development of crypts [5] , [6] , [7] . In the list of upregulated genes in the middle intestine of Blimp1 mutant animals, we observed a significant amount of Paneth cell-specific genes at P7 such as lysozyme and a number of α-defensins ( Fig. 8a ). We therefore performed immunohistochemical staining for lysozyme, which specifically marks lysosomal granules of mature Paneth cells and found that Blimp1 mutant animals had accelerated Paneth cell development ( Fig. 8b,c ). This phenotype was especially clear in the distal small intestine where only 18% of crypts contained Paneth cells in wild-type mice ( n =9), but 100% of crypts contained Paneth cells in Blimp1 mutant mice ( n =6). This gave further confirmation of the enhanced crypt maturation in Blimp1 mutant animals. As we found an increase in the number of Paneth cells in the mutant mice, we also studied the presence of the other two secretory lineages. Goblet cells were identified using a periodic acid-Schiff stain, whereas the enteroendocrine cells were detected using immunohistochemistry for synaptophysin [45] . This analysis showed a modest increase of the number of goblet cells without the regional difference that was observed for the Paneth cells ( Fig. 8d,e ). No change was observed in the number of enteroendocrine cells, which was very low in both wild types and Blimp1 mutants ( Fig. 8f,g ). 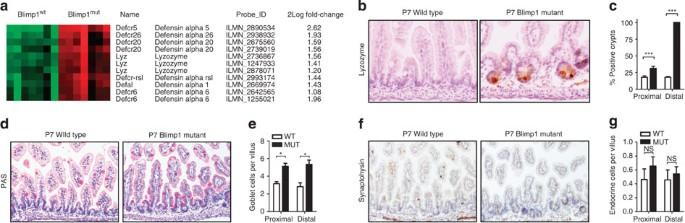Figure 8: Premature development of Paneth cells in Blimp1 mutant (MUT) mice. (a) Heatmap of specific Paneth cell genes that are upregulated in the mid-intestine of the Blimp1 MUT animals. (b) Immunohistochemistry for lysozyme shows premature presence of Paneth cells in Blimp1 MUT animals at P7. Original magnification ×400. (c) The percentage of crypts containing Paneth cells was larger in MUT mice than in wild types (WTs), with the most remarkable difference in the distal small intestine, ***P<0.001, two-way analysis of variance. (d) Periodic acid-Schiff (PAS) staining shows goblet cells in the distal intestine of WT and Blimp1 MUT mice. (e) Quantification of the number of PAS-positive goblet cells per villus in the proximal (3.2±0.25 versus 5.1±0.34 in WT versus MUT) and distal intestine (2.8±0.38 versus 5.3±0.53 in WT versus MUT). (f) Immunohistochemistry for synaptophysin in WT and Blimp1 MUT mice. (g) Quantification of the number of synaptophysin-positive enteroendocrine cells per villus in the proximal (0.46±0.18 versus 0.67±0.13 in WT versus MUT) and distal intestine (0.46±0.14 versus 0.54±0.10 in WT versus MUT). *P<0.05, two-way analysis of variance. Original magnifications ×200. NS, not significant. Figure 8: Premature development of Paneth cells in Blimp1 mutant (MUT) mice. ( a ) Heatmap of specific Paneth cell genes that are upregulated in the mid-intestine of the Blimp1 MUT animals. ( b ) Immunohistochemistry for lysozyme shows premature presence of Paneth cells in Blimp1 MUT animals at P7. Original magnification ×400. ( c ) The percentage of crypts containing Paneth cells was larger in MUT mice than in wild types (WTs), with the most remarkable difference in the distal small intestine, *** P <0.001, two-way analysis of variance. ( d ) Periodic acid-Schiff (PAS) staining shows goblet cells in the distal intestine of WT and Blimp1 MUT mice. ( e ) Quantification of the number of PAS-positive goblet cells per villus in the proximal (3.2±0.25 versus 5.1±0.34 in WT versus MUT) and distal intestine (2.8±0.38 versus 5.3±0.53 in WT versus MUT). ( f ) Immunohistochemistry for synaptophysin in WT and Blimp1 MUT mice. ( g ) Quantification of the number of synaptophysin-positive enteroendocrine cells per villus in the proximal (0.46±0.18 versus 0.67±0.13 in WT versus MUT) and distal intestine (0.46±0.14 versus 0.54±0.10 in WT versus MUT). * P <0.05, two-way analysis of variance. Original magnifications ×200. NS, not significant. Full size image Thus, Blimp1 is not only just a regulator of enterocyte specialization but also seems to affect the maturation of the intestinal epithelium at a more global level. The intestinal epithelium of the suckling neonate has a number of morphological and metabolic features that allow optimal processing of mother's milk [1] . These features are lost at the suckling to weaning transition when the intestinal epithelium adapts to major changes in diet and undergoes final maturation. It has previously been shown that these important epithelial maturation stages depend on factors that are intrinsic to the intestine and occur normally independent of specific luminal or extraintestinal influences [15] , [16] , [17] . The nature of the intrinsic regulators remained elusive to date. In the current study, we find that Blimp1 is expressed in the developing and postnatal intestinal epithelium, and that expression is specifically lost at the suckling to weaning transition. Intestine-specific deletion revealed that Blimp1 controls multiple aspects of the maturation of the suckling-type neonatal epithelium to the adult-type epithelium. The neonatal intestine has several features that are distinct from the fully mature intestinal epithelium of the adult mouse. These features seem to make the epithelium especially prepared to absorb and digest the high-fat, low-carbohydrate diet of milk, which contains lactose as a major source of carbohydrates [1] . The neonatal epithelium has a highly developed apical canilicular system at the cell surface. The canaliculi feed luminal immunoglobulins and other macromolecules from milk into large intracellular vacuoles and facilitate the transport of these molecules across the epithelial barrier without loss of biological activity [2] , [3] . The brush border of the neonate is not as well developed as the brush border of the adult enterocyte and contains lactase as the major disaccharidase to digest the lactose present in milk [1] . Our current studies identified another disaccharidase with the potential to metabolize lactase as specific for the normal neonatal epithelium. We found that the enterocytes express β-galactosidase in the cytoplasmic vacuoles in this period [33] , [34] . In contrast, after the suckling period, the brush border is better developed and contains sucrase isomaltase, a disaccharidase that can digest fructose and more complex carbohydrates. Another feature of the neonatal epithelium is related to the low concentrations of arginine in milk and the requirement of arginine for growth during the neonatal period. Neonatal enterocytes can synthesize arginine from its precursors glutamine and proline that are abundantly present in milk. For this arginine synthesis, one of the critical intermediate steps is the generation of argininosuccinate from citrulin by argininosuccinate synthetase 1 (ref. 38 ). On the other hand, neonatal enterocytes lack the expression of arginase, which is typical for adult intestinal epithelial cells, probably to minimize intestinal catabolism of arginin and maximize output to the blood stream [39] , [40] , [41] , [42] . Our studies showed that all of these specific adaptations of neonatal intestinal epithelium were absent in Blimp1 mutant mice. The strongly reduced neonatal fitness with excess postnatal mortality and severe growth retardation in the surviving mutant mice clearly shows the importance of the specific epithelial phenotype in processing mother's milk during the suckling period. Many of the 145 upregulated genes in the gene array were implicated in metabolic pathways. For example, 40 of these genes have a role in lipid metabolism, small molecule biochemistry and transport. That is consistent with differentially expressed protein sets previously reported in a proteome analysis of the mouse from suckling to weaning transition [27] . Significantly, our gene list showed that our Blimp1 mutant mice recapitulate some of the individual enzymatic changes, which are normally found to occur from the suckling to weaning transition in this proteome analysis. For example, it was found in the proteome analysis that alcohol dehydrogenase 1 was upregulated at the suckling to weaning transition and we found alcohol dehydrogenase 1 among the upregulated genes in our mutant mice. Similarly, it was found that sialidase-1 (Neu1) is normally downregulated at the suckling to weaning transition and we find that it is lost in our mutant mice. Similarly, Mochizuki et al . [46] studied gene expression changes in the jejunum of rats at suckling to weaning transition and identified many genes upregulated at this developmental time point that are also significantly upregulated in our mutant mice such as Slc13a2 , Aqp3 , Slc4a1 , Abcg8 , Abcg5 , Rdh7 , Cyp4f , Aldh1a7 , Dpep1 and Adh4 . On the other hand, some of the genes that were identified by Mochizuki et al . [46] as downregulated at the suckling to weaning transition such as Nox4 , Folr1 and Neu1 were also downregulated in Blimp1 mutants. This is further evidence that transformation of suckling-type intestinal epithelium to adult-like epithelium had occurred at a global genomic scale. Furthermore, the fact that our real-time RT–PCR showed that the adult-type enzymes were already derepressed at E17.5 is clear evidence of the fact that the expression of such enzymes can be established completely independent of luminal or extraintestinal factors. Blimp1 mutant mice have enhanced formation of crypts at P7. Postnatal crypt formation is a poorly studied phenomenon. A careful morphological analysis has shown that the distance between the base of the intervillus epithelium and the circular smooth muscle layer remains constant during crypt formation [28] . Crypt formation seems to involve mesenchymal enveloping of the nascent crypt and upwards migration of the crypt–villus junction [28] . As loss of Blimp1 results in major alterations in the epithelial cells on the villus, this may affect crypt formation indirectly, via effects on the mesenchyme. This would be in accordance with the fact that we do not observe major changes in the expression of Ki67, c-Myc or Sox9, and did not find major alterations in genes associated with precursor cell phenotype in the gene array. However, as Blimp1 is expressed in the prospective crypt cells until around P0, an alternative explanation may be that the crypt cells were affected by the loss of Blimp1 at an earlier time point in development. Another aspect of the premature phenotype of the Blimp1 mutant intestine was the accelerated formation of Paneth cells, which normally appears coincident with crypt formation between P7 and P28 (ref. 5 ). Loss of Blimp1 only modestly affected the number of goblet cells and did not affect the number of enteroendocrine cells. This argues against an effect on common regulators of the development of the secretory lineage such as Wnt signalling [45] , Hes1 (ref. 47 ) or Math1 (ref. 48 ). Further experiments will be required to address the link between Blimp1 and Paneth cells. A further phenotype we identified in the Blimp1 mutant mice is accelerated epithelial migration. This is another change that is known to develop only around the suckling to weaning transition [5] . Thus, Blimp1 is responsible for a global delay in intestinal epithelial maturation that affects multiple aspects of the intestinal phenotype. While this manuscript was in preparation, a study by Harper et al . [49] with similar findings to our own was published. The authors also observed the rapid decline in Blimp1 in the postnatal intestine and also created a VillinCre-Blimp1 conditional mutant. Harper et al. [49] made many observations that concur with our own findings and even identified many of the same changes of enzyme expression in the global analysis of gene expression. The major difference between our and their studies is that Harper et al . [49] do not describe the accelerated crypt formation and some of the features that were most clear in or specific for the distal small intestine, such as the early formation of Paneth cells and the disappearance of the cytoplasmic vacuoles in the mutant mice. These features may depend on the background of the mice, the environment in which they are housed and/or the segment of intestine that was examined. In conclusion, we find that the transcriptional repressor Blimp1 is specifically expressed in the developing and postnatal intestine, and that Blimp1 is required to delay final maturation of the intestinal epithelium to the suckling to weaning transition. Mice Blimp1 fl/fl18 , VillinCre [26] transgenic and Cyp1a1Cre [50] mice have previously been described. We generated VillinCre + Blimp1 fl/fl animals, resulting in intestine-specific Blimp1 deletion from around E14.5. Mice were bred as breeding pairs that were heterozygous for the Blimp1 floxed allele. The initial VillinCre + Blimp1 fl/fl (Blimp1 mutant), VillinCre + Blimp1 +/+ and VillinCre − Blimp1 fl/fl (Blimp1 wild type) offspring was used for the gene array analysis. From the fourth generation of crosses onward, the VillinCre transgene was inbred and no Cre -negative animals were observed. These mice were used for the analysis of the Mendelian ratio at birth and neonatal survival. Mice were collected at different stages: E17.5, just before birth (P0), P7, P14, P21 and week 6 after birth. To conditionally delete Blimp1 in the adult small intestinal epithelium, Blimp1 fl/fl were crossed with Cyp1a1Cre mice. At 6 weeks of age, Cyp1a1Cre + Blimp1 fl/fl mice received intraperitoneal injections with either 80 mg kg −1 β-naphthoflavone (Sigma) or vehicle (corn oil) for 5 days in a row. All animals were housed in the Leiden University Medical Center's experimental animal centre. All the experiments were approved by the Institutional Animal Care and Use Committee of the University of Leiden. Histology and immunohistochemistry Tissue was fixed overnight in 4% formaldehyde, embedded in paraffin and sectioned. For immunohistochemistry, sections were deparaffinized using xylene and rehydrated in a series of ethanols. Endogenous peroxidases were blocked using methanol with 3% H 2 O 2 . For antigen retrieval, tissue was boiled at 100 °C on a heat block in 0.01 M EDTA (pH 9) for 20 min. Subsequently, slides were incubated with a primary antibody in PBS with 1% bovine serum albumin and 0.1% Triton X-100. Sections were then washed and incubated with a Powervision secondary antibody (Immunologic) for 1 h. Slides were washed in PBS. The chromagen substrate consisted of diaminobenzedine (Sigma), and was used according to the manufacturer's instructions. For immunohistochemistry of Blimp1, we used a rat monoclonal anti-Blimp1 (1:250, clone 6D3, sc-47732, Santa Cruz). The specificity of this antibody for Blimp1 was confirmed by loss of epithelial Blimp1 expression in the mutant mice and by western blot of Blimp1-transfected HCT116 cells ( Supplementary Fig. S4 ). Other antibodies used were: a rabbit polyclonal anti-adenosine deaminase (1:250, H-300, sc-25747, Santa Cruz), a rabbit polyclonal anti-trehalase (1:250, GTX109979, GeneTex), rabbit polyclonal anti-argininosuccinate synthetase 1 (1:2000) [51] , mouse monoclonal anti-beta-galactosidase (1:500, Z3783, Promega), a goat polyclonal anti-sucrase isomaltase (1:250, A17, sc27603, Santa Cruz), a rabbit polyclonal anti-lactase (1:500) was a kind gift from Dr K.-Y.Yeh [52] , a rabbit polyclonal anti-c-Myc (1:500, N-262, sc-764, Santa Cruz), a rabbit polyclonal anti-Sox9 (1:700, AB5535, Millipore), a mouse monoclonal anti-Cdx2 (1:250, MU382A-UC, Biogenex) and a rabbit polyclonal anti-synaptophysin (1:50, A0010, DAKO). RNA studies Intestinal tissue was homogenized in 1 ml Trizol (Invitrogen) and RNA extraction was performed according to the manufacturer's instructions. For cDNA synthesis, 1 μg of RNA was transcribed using Revertaid (Fermentas). Real-time RT–PCR was performed using SybrGreen (Qiagen) according to the manufacturer's protocol on a BioRad iCycler using following primers (AdaI fw : 5′-GACACCCGCATTCAACAAAC-3′, AdaI rev : 5′-ATGCCTCTCTTCTTGCCAAA-3′, ArgII fw : 5′-TGATTGGCAAAAGGCAGAGG-3′, ArgII rev : 5′-CTAGGAGTAGGAAGGTGGTC-3′, AssI fw : 5′-CATTGGAATGAAGTCCCGAG-3′, AssI rev : 5′-GATTTTGCGTACTTCCCGAT-3′, Cyclophilin fw : 5′-ATGGTCAACCCCACCGTGT-3′, Cyclophilin rev : 5′-TTCTGCTGTCTTTGGAACTTTGTC-3′, Glb1 fw : 5′-ACTGCTGCAACTGCTGGG-3′, Glb1 rv : 5′-AATGGCTGTCCATCCTTGAG-3′, SI fw : 5′-GCCCACGCGTTTGGTGAGAC-3′, SI rev : 5′-ATCAGCAGTGCAGGGCCCCA-3′, Treh fw : 5′-GCACCTGCTGCTTCTGCT-3′, Treh rv : 5′-CATCTGAACTTGGTGCAGGA-3′). For microarray analysis, RNA from the whole mid-intestine was purified using Trizol (Invitrogen) according to the manufacturer's instructions. RNA was cleaned through an RNEasy column (Qiagen). Total RNA (150 ng) was labelled using the cRNA labelling kit for Illumina BeadArrays (Ambion) and hybridized with Ref8v3 BeadArrays (Illumina). Arrays were scanned on a BeadArray 500GX scanner. Using GenomeStudio software (Illumina), arrays were normalized using quantile normalization and the background was subtracted. All genes that had negative values only were removed from analysis. Differentially expressed genes were extracted using remote analysis computation for gene expression data. Differentially expressed genes had a P -value <0.05 (analysis of variance), followed by an false discovery rate post analysis correction for multiple comparisons. The Geo accession number for the array data is: GSE30556 . Heatmaps were generated using TreeView software. Transmission electron microscopy Small intestine was dissected and from the ileum a small piece of tissue, about 3 mm long, was cut out. After fixation, the material was postfixed in 1% osmium tetroxide, with block staining with 1% uranyl acetate, one-step dehydration in dimethoxypropane and embedding in epoxy resin LX-112. Sections were stained with tannic acid, uranyl acetate and lead citrate, and examined in a transmission electron microscope (FEI/Philips CM10). Acccession codes: The microarray data has been deposited in the GEO database under the accession code GSE30556 . How to cite this article: Muncan, V. et al . Blimp1 regulates the transition of neonatal to adult intestinal epithelium. Nat. Commun. 2:452 doi: 10.1038/ncomms1463 (2011).